Regulation of the co-evolved HrpR and HrpS AAA+ proteins required forPseudomonas syringaepathogenicity The bacterial AAA+ enhancer-binding proteins (EBPs) HrpR and HrpS (HrpRS) of Pseudomonas syringae ( Ps ) activate σ 54 -dependent transcription at the hrpL promoter; triggering type-three secretion system-mediated pathogenicity. In contrast with singly acting EBPs, the evolution of the strictly co-operative HrpRS pair raises questions of potential benefits and mechanistic differences this transcription control system offers. Here, we show distinct properties of HrpR and HrpS variants, indicating functional specialization of these non-redundant, tandemly arranged paralogues. Activities of HrpR, HrpS and their control proteins HrpV and HrpG from Ps pv. tomato DC3000 in vitro establish that HrpRS forms a transcriptionally active hetero-hexamer, that there is a direct negative regulatory role for HrpV through specific binding to HrpS and that HrpG suppresses HrpV. The distinct HrpR and HrpS functionalities suggest how partial paralogue degeneration has potentially led to a novel control mechanism for EBPs and indicate subunit-specific roles for EBPs in σ 54 -RNA polymerase activation. Many bacterial pathogens use a type-three secretion system (T3SS) to deliver proteins into host cells (reviewed in ref. 1 ). hrp and hrc genes establish the regulatory and structural functions associated with the T3SS from the group I-type hrp / hrc cluster of Pseudomonas , Erwinia and former Erwinia phytopathogens (for example, Pectobacterium and Dickeya spp.) [2] . hop genes encode secreted pathogenicity effectors and the majority of hop genes and hrp / hrc cluster genes are regulated by the extracytoplasmic function σ-factor HrpL, which is regulated by the σ 54 -dependent hrpL promoter [3] , [4] . Regulation of σ 54 -RNA polymerase (σ 54 -RNAP) activity is achieved by the action of specific enhancer-binding proteins (EBPs) [5] , [6] . In phytopathogenic fluorescent Pseudomonas spp., other than Pseudomonas syringae ( Ps ), and in the phytopathogenic species in the Enterobacteriaceae, a single EBP, HrpS, activates transcription from the hrpL promoter [7] . In Ps, hrpL expression is activated by a co-dependent pair of EBPs; HrpR and HrpS [8] . EBPs are molecular machines belonging to the AAA+ ( A TPases a ssociated with various cellular a ctivities) superfamily [9] of P-loop ATPases. They remodel σ 54 -RNAP at its promoter sites and, via a carboxy (C)-terminal HTH domain, bind promoter upstream activator sites (UASs). The ATPase activity of EBPs relies on the formation of hexameric ring-like assemblies [6] . This feature is commonly exploited by cis -acting regulatory domains to control the activity of EBPs by either impairing (as in DctD and NtrC1) or promoting (as in NtrC) hexamer assembly [10] . The EBPs HrpR and HrpS, similar to the well-studied EBP PspF, lack cis -acting regulatory domains and comprise only the AAA+ and HTH domains. PspF activity is directly negatively regulated by an additional protein, PspA [11] . HrpV is thought to fulfill a similar regulatory role in the HrpRS and probably HrpS systems [12] . Repression of HrpV is proposed to be released through the action of HrpG [13] . The vast majority of bacterial AAA+ proteins studied so far form homo-hexameric AAA+ rings, whereas their eukaryotic isoenzymes often function as heteromeric assemblies. For instance, the mini chromosomal maintenance (MCM) complex, a processive replicative helicase, functions as a typical AAA+ homo-hexameric ring in archaea [14] , but the eukaryotic isoenzyme (MCM: Mcm2-7p) is heteromeric [15] . The hrpRS genes are transcribed as an operon, proposed to form a functional heteromeric HrpRS AAA+ complex of unknown quaternary structure [8] . The advantage that such a dual EBP system confers on T3SS-mediated pathogenicity in Ps is unclear. Multiple sensory systems as well as abiotic and biotic inputs are used in regulating expression from group I hrp regulons. Among these sensory systems are Lon, GacA, HrpXY, rsmA/B, HrpRS, HrpV, HrpG and quorum-sensing components [7] , [8] , [12] , [13] , [16] , [17] , [18] , [19] . Here, we study the HrpRS, HrpV and HrpG components of Ps DC3000 and report: direct evidence for a single mixed composition functional hexameric HrpRS complex; that HrpR and HrpS each contact σ 54 ; that HrpR and HrpS make unequal contributions to the ATP-dependent and HrpV-controlled functioning of the hetero-hexamer and; specific binding of HrpV to HrpS is used in a novel inhibition and regulation mechanism that is sensitive to HrpG action. These findings provide detailed insights into the molecular evolution of an EBP system that distinguishes Ps from non- syringae plant pathogens. Gene duplication leading to HrpRS is distinctive for Ps In Ps (including DC3000), hrpR and hrpS are arranged in tandem ( hrpRS ), transcribed as a single operon [8] and exhibit high sequence similarity, suggesting that they have evolved from a single ancestral gene duplication event. A search for the highest similar sequences for group I-type pathogenicity islands (PAIs) identified ten non-redundant hrpRS tandem arrangements (in Ps pathovars) and ten single- hrpS sequences (in Erwinia -type pathovars as well as the hrpS homologue rspR from P. fluorescens ). All 20 inspected PAIs also harbour the regulatory genes hrpV and hrpG , including P. mendocina (a P. aeruginosa -related human pathogen [20] ), suggesting that the appearance of hrpRS is more recent than that of the presumed hrpS regulatory genes (hrpV and hrpG ). Although regulatory roles for HrpV and HrpG remain to be established for non- syringae strains they have been clearly annotated as hrpV and hrpG across genera and the synteny of the intra-operon loci are strictly conserved. A phylogenetic tree based on protein sequences derived from the 30 EBPs obtained is shown in Supplementary Figure S1 . Where present HrpR and HrpS have 55–65% sequence identity and 70–79% sequence similarity to each other ( Supplementary Table S1 —compared with other well-studied bacterial EBPs, such as ZraR, PspF, NtrC1, which have 38–41% identity; Supplementary Table S2 ). Strikingly, hrpRS was found in all Ps pathovars, making the dual hrpRS EBP system a distinguishing feature in the hrp/hrc gene cluster of group I PAI in Ps pathovars. Further, no polymorphism ( hrpRS or hrpS ) has been reported for Ps . We did not find polymorphism among identified PAI (including among redundant sequences); strongly suggesting that hrpRS in Ps provides a selective advantage compared with singly acting hrpS. The exact branch pattern symmetry between the HrpS RS and HrpR groups ( Supplementary Fig. S1 ) suggests that following gene duplication, hrpR and hrpS may not have diverged freely as is commonly assumed in gene duplication due to functional redundancy [21] , [22] . Inspection of the HrpR and HrpS sequences of Ps DC3000 and their predicted structures indicate no obvious basis of their co-dependency. They show clear congruence with other EBPs ( Supplementary Fig. S2 ), in that the seven conserved regions identified for all EBPs and the conserved AAA+ motifs are present ( Fig. 1a ) [5] . 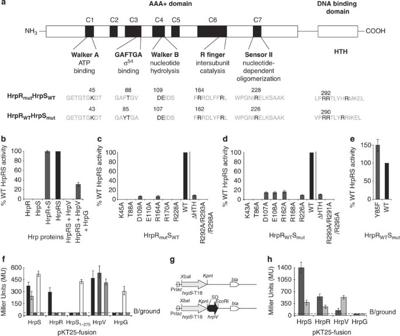Figure 1:In vivotranscription and protein–protein interactions of Hrp proteins. (a) Domain organization of EBPs showing the seven conserved regions (C1–C7) and their associated functions. HrpR and HrpS key motif sequences are given with the sites of amino-acid substitutions (used inc,d,ebelow) indicated (black typeface numbering refers to amino-acid position in either HrpR or HrpS). (b)In vivotranscription activation activities measured from the chromosomal promoterhrpL∷lacZreporter construct—given as a percentage of WT co-expressed (single operon) HrpRS activity (where WT=100%)—of singly expressed HrpR or HrpS, and co-expressed HrpR+HrpS (HrpR+S) (from different plasmids). HrpV expression abolishes HrpRSin vivoactivity (HrpRS+HrpV), which is partly relieved when co-expressing HrpG (HrpRS+HrpV+HrpG). (c) As inbtranscription activation by HrpRS, where HrpR carries mutations as indicated. (d) As inbtranscription activation by HrpRS, where HrpS carries mutations as indicated. (e) As inbtranscription activation by HrpRS, where HrpS carries the gain of function mutation Y85F. (f) Bar graph depicting results of the BACTH protein–protein binding interactions between HrpR (black), HrpS (light grey), HrpS1−275(dark grey), HrpV (white), HrpG (grey) inferred by β-galactosidase production and displayed in Miller Units (MU)32. B/ground represents the background level of β-galactosidase activity detected for the negative control (30 MU—obtained with the two-hybrid vectors in the absence of protein fusions). (g) Scheme of the expression construct for the BACTH three component system. (h) Bar graph depicting the binding interactions between T25-fused proteins HrpR, HrpS, HrpV and HrpG with T18C-fused HrpS in the presence of co-expressed HrpV in a three-component two-hybrid system35inferred by β-galactosidase production and displayed in Miller Units. Inb–e, all assays were minimally performed in triplicate and standard errors of the mean are shown. Protein expression was verified by western blotting (seeSupplementary Fig. S3). Figure 1: In vivo transcription and protein–protein interactions of Hrp proteins. ( a ) Domain organization of EBPs showing the seven conserved regions (C1–C7) and their associated functions. HrpR and HrpS key motif sequences are given with the sites of amino-acid substitutions (used in c , d , e below) indicated (black typeface numbering refers to amino-acid position in either HrpR or HrpS). ( b ) In vivo transcription activation activities measured from the chromosomal promoter hrpL ∷ lacZ reporter construct—given as a percentage of WT co-expressed (single operon) HrpRS activity (where WT=100%)—of singly expressed HrpR or HrpS, and co-expressed HrpR+HrpS (HrpR+S) (from different plasmids). HrpV expression abolishes HrpRS in vivo activity (HrpRS+HrpV), which is partly relieved when co-expressing HrpG (HrpRS+HrpV+HrpG). ( c ) As in b transcription activation by HrpRS, where HrpR carries mutations as indicated. ( d ) As in b transcription activation by HrpRS, where HrpS carries mutations as indicated. ( e ) As in b transcription activation by HrpRS, where HrpS carries the gain of function mutation Y85F. ( f ) Bar graph depicting results of the BACTH protein–protein binding interactions between HrpR (black), HrpS (light grey), HrpS 1−275 (dark grey), HrpV (white), HrpG (grey) inferred by β-galactosidase production and displayed in Miller Units (MU) [32] . B/ground represents the background level of β-galactosidase activity detected for the negative control (30 MU—obtained with the two-hybrid vectors in the absence of protein fusions). ( g ) Scheme of the expression construct for the BACTH three component system. ( h ) Bar graph depicting the binding interactions between T25-fused proteins HrpR, HrpS, HrpV and HrpG with T18C-fused HrpS in the presence of co-expressed HrpV in a three-component two-hybrid system [35] inferred by β-galactosidase production and displayed in Miller Units. In b – e , all assays were minimally performed in triplicate and standard errors of the mean are shown. Protein expression was verified by western blotting (see Supplementary Fig. S3 ). Full size image Specialization of HrpR and HrpS mechanism and regulation Initially, we expressed wild-type (WT) HrpR, HrpS, HrpV and HrpG in Escherichia coli , and assayed activities using a P hrpL ∷ lacZ reporter integrated into the chromosome (see Methods and Supplementary Table S3 ). As shown in Figure 1b , co-expressed HrpR and HrpS (expressed simultaneously from different plasmid constructs) or HrpRS (co-expressed as a single operon), but not HrpR or HrpS alone (expressed singly), resulted in elevated β-galactosidase activity—in line with the strict requirement for both HrpR and HrpS to activate hrpL transcription. Western blotting confirmed that both HrpR and HrpS were stably expressed, excluding gross protein instability at the level of proteolysis as a basis of their co-dependence in vivo ( Supplementary Fig. S3 ), although HrpR–HrpS assembly defects cannot be excluded. Co-expression of HrpRS and HrpV resulted in reduced transcription activation ( Fig. 1b , HrpRS+HrpV), demonstrating that HrpV negatively controls the functionality of HrpRS in the absence of other Ps -specific factors in vivo . Notably, expression of HrpG partly released the negative effect of HrpV on HrpRS activity. Biochemical studies with AAA+ proteins, including EBPs, suggest that non-synchronized ATP hydrolysis occurs between individual subunits of homomeric complexes [23] , [24] . To address this notion more directly, we introduced equivalent single amino-acid substitutions into EBP functionally important motifs in either HrpR or HrpS ( Fig. 1a ) to delineate the specific roles of conserved EBP sequences within the context of heteromeric HrpRS [6] . We assayed the effect of amino-acid substitutions, on in vivo P hrpL transcription activation ( Fig. 1c,d ). As shown in Figure 1c,d , the β-galactosidase activities of HrpR and HrpS variant forms demonstrated that the integrity of the Walker A (P-loop) motif was required for in vivo promoter activation. Substitutions in the HrpS Walker B motif (E108, Fig. 1d ), expected to be essential for ATP hydrolysis, and the sensor II residue R226, retain significant residual activity (51 Miller Units (MU) and 32 MU, respectively). In contrast ( Fig. 1c ) the corresponding substitutions in HrpR showed no detectable activity (E110 and R228; 2 MU and 1 MU, respectively; where the background level is 2 MU and 100% activity corresponds to 350 MU). Given that Walker B residues and the sensor II 'R' residue are critical for ATP hydrolysis and EBP functionality (in terms of the ability to stimulate open complex (OC) formation) [25] , [26] , these data suggest mechanistic subunit specialization in the ATP hydrolysis-associated functionalities of HrpR and HrpS. EBPs contact σ 54 via the consensus GAFTGA motif [27] . Such interactions depend on the nucleotide-bound state [28] , [29] , [30] and rely on the integrity of the 'F' and 'T' residues [27] , [31] . In HrpR, this sequence is predominantly GAFTGV and in HrpS is always GAYTGA (including in singly acting HrpS; Supplementary Fig. S2 ). Deviation from the consensus GAFTGA motif in HrpR and HrpS may reflect subunit specialization in contacting σ 54 . Substituting Y for F in HrpS, resulted in a 50% increase in activity compared with WT HrpRS ( Fig. 1e ), indicating that HrpS can interact with σ 54 , yet appears to limit the activity of HrpRS. As substituting Y for F in HrpS did not overcome the requirement for HrpR, we infer that the non-consensus residue Y85 is not the basis of HrpRS co-dependency. Substitution of the near invariant T residue (present in >97% of identified EBPs; a key σ 54 -contacting residue, yet does not affect the self-assembly or ATPase activities of PspF [27] ) for A in either HrpR or HrpS led to a loss of transcription activation; demonstrating that both the HrpR and HrpS σ 54 -contacting 'GAFTGA' sequences are strictly required. Clearly HrpR and HrpS have each evolved mechanistic specialization, providing direct evidence for subunit-specific roles of this novel EBP system in activating σ 54 -RNAP. Interactions between the Hrp proteins We analysed the protein–protein interactions that occur within the HrpRS, HrpV and HrpG regulatory complexes in vivo using a bacterial two-hybrid system, BACTH [32] . We verified that all two-hybrid fusion proteins were similarly expressed ( Supplementary Fig. S3 )—thereby establishing that failure to detect an interaction was not simply due to unstable Hrp-fusion proteins. Consistent with earlier findings, HrpS self-associates and interacts with both HrpR and HrpV, but not HrpG ( Fig. 1f ). HrpV also interacts with HrpG. HrpR did not detectibly interact with itself, HrpV or HrpG ( Fig. 1f and refs 8 , 13 ). Glutaraldehyde crosslinking with co-purified HrpRS and purified HrpV, and followed by western blotting using antibodies specific to HrpR, HrpS (His-tag) and HrpV established direct binding of HrpV to HrpS can occur independently of additional factors ( Supplementary Fig. 3 ). To distinguish which HrpS domain contributed to the different binding interactions, we created a C-terminal HTH truncation variant, HrpS 1−275 (the HrpS AAA+ domain), and analysed interactions with full-length (FL) HrpS, HrpR, HrpV and HrpG. In contrast to HrpS, HrpS 1−275 showed no detectable interactions with itself or HrpR—suggesting oligomerization determinants in HrpS reside in the HTH domain, consistent with dimerization functionalities in NtrC [33] . Importantly, interaction activities are retained between HrpS 1−275 and HrpV, suggesting that HrpV acts directly by binding the HrpS AAA+ domain. Regulation of EBPs is commonly achieved by altering higher-order oligomer formation (and hence ATPase activity [10] , [34] ). We therefore tested whether HrpV affected subunit-binding interactions within the HrpRS complex by co-expressing native HrpV together with the BACTH protein fusions to form a three-component system ( Fig. 1g ) [35] . Our results demonstrate that expression of native HrpV greatly increased HrpS self-association and moderately increased HrpR–HrpS interactions ( Fig. 1h ), suggesting that HrpV binding to HrpS somewhat alters subunit–subunit interactions within the self-assembled HrpRS complex. Western blotting confirmed that the levels of HrpR and HrpS production were similar in the presence of the extra copy of HrpV ( Supplementary Fig. S3 ). Given the absence of detectable interactions between HrpS and HrpG (even in the presence of HrpV), we infer that HrpV may not bind HrpS and HrpG simultaneously and that HrpG relieves HrpV inhibition by precluding HrpV–HrpS interactions. HrpV and HrpG act antagonistically to control HrpRS activity The ways in which heteromeric EBPs may differ from singly acting EBPs are not known. We therefore investigated features in the HrpRS system that are common to EBPs: the presence of and co-operative binding to UAS DNA; a facilitating role of integration host factor (IHF) to increase productive interactions between the EBP and σ 54 -RNAP closed complex; a strict nucleotide-dependency during transcription activation, and the regulation of EBPs by modulating the oligomeric state and/or DNA-binding activity. To gain insights into the HrpRS system, we purified FL HrpR, HrpS, HrpRS (co-expressed), IHF, HrpV and HrpG. In vitro studies of many other EBPs [36] , [37] have been performed using isolated EBP domains, because of the difficulties associated with limited solubility of FL EBPs [38] , [39] , [40] , [41] . HrpR and HrpS when expressed and purified separately resulted in substantially lower protein yields than co-expressed HrpRS, suggesting that HrpR/HrpS mutually stabilize a soluble heteromeric conformation (in line with oligomerization determinants residing within the AAA+ and HTH domains; Fig. 1c,d,f ). Further, attempts to co-purify HrpRS complexes harbouring Walker B alanine substitutions in either HrpR or HrpS resulted in very low protein yields, probably due to a failure to form stable HrpRS complexes as observed with the equivalent substitutions in PspF [42] . The activity of the purified HrpRS complex was measured using an in vitro single-round transcription assay from the supercoiled hrpL promoter. 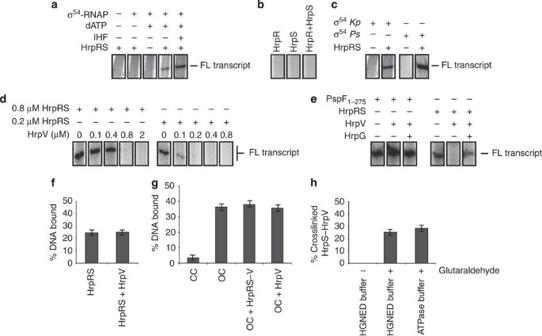Figure 2: Regulation of the HrpRS complexin vitro. (a)In vitrofull-length (FL) transcription assays (∼470 nucleotides) using the supercoiledhrpLpromoter in the presence (+) or absence (−) of: σ54-RNAP (100 nM), dATP (4 mM), co-purified HrpRS (0.8 μM) and integration host factor (IHF) (20 nM). (b) HrpR alone (0.8 μM), HrpS alone (0.8 μM) and pre-mixed HrpR and HrpS (0.8 μM) (HrpR+HrpS) failed to activate transcription. (c) As ina, including dATP (4 mM), IHF (20 nM) with reconstituted σ54-RNAP using either purified σ54fromPs(σ54-Ps) or from σ54K. Pneumoniae(σ54-Kp). (d) HrpRS-dependent activation from thehrpLpromoter as ina, in the presence of increasing HrpV concentrations. (e) Transcription from a test σ54promoter (S. meliloti nifH), with the EBP AAA+ domain PspF1−275, or HrpRS, and in the presence (+) or absence (−) of HrpV (2 μM) and HrpG (2 μM). Gel images of transcripts forFigure 2a–eare shown inSupplementary Figure 4. (f) A bar graph showing electrophoretic mobility shiftedhrpLDNA promoter probe comprising UAS sequences (in percentage of totalhrpLDNA promoter signal) in the presence of HrpRS (2.5 μM) or HrpRS (2.5 μM and HrpV (4.2 μM). (g) A bar graph depicting the percentage of DNA bound in the closed promoter complex (CC) and transcriptionally proficient open promoter complex (OC; formed by PspF activation) in the presence of HrpRS–V or HrpV. (h) A bar graph depicting the relative amount of glutaraldehyde crosslinked HrpRS–HrpV species in either ATPase buffer (used to measure the ATPase activity of HrpRS+/−HrpV) or HGNED buffer. The relative amount of crosslinked HrpS–V complex was determined by fluorescence scanning. Inf–h, estimated errors of measurements are shown as ±10%. As shown in Figure 2a , FL transcript formation required σ 54 -RNAP, dATP and HrpRS. Purified IHF greatly stimulated the amount of FL transcript obtained in vitro . Notably, the absence of FL transcripts with HrpR alone, HrpS alone or separately purified and mixed in vitro HrpR and HrpS (HrpR+HrpS), suggests that in vivo self-assembly of the HrpRS complex is important for forming the active HrpRS complex ( Fig. 2b ). HrpRS activated transcription when RNAP was reconstituted with either Klebsiella pneumoniae ( Kp ) or Ps σ 54 ( Fig. 2c ), indicating that HrpRS can function independently of Ps -specific σ 54 . Figure 2: Regulation of the HrpRS complex in vitro . ( a ) In vitro full-length (FL) transcription assays ( ∼ 470 nucleotides) using the supercoiled hrpL promoter in the presence (+) or absence (−) of: σ 54 -RNAP (100 nM), dATP (4 mM), co-purified HrpRS (0.8 μM) and integration host factor (IHF) (20 nM). ( b ) HrpR alone (0.8 μM), HrpS alone (0.8 μM) and pre-mixed HrpR and HrpS (0.8 μM) (HrpR+HrpS) failed to activate transcription. ( c ) As in a , including dATP (4 mM), IHF (20 nM) with reconstituted σ 54 -RNAP using either purified σ 54 from Ps (σ 54 - Ps ) or from σ 54 K. Pneumoniae (σ 54 - Kp ). ( d ) HrpRS-dependent activation from the hrpL promoter as in a , in the presence of increasing HrpV concentrations. ( e ) Transcription from a test σ 54 promoter ( S. meliloti nifH ), with the EBP AAA+ domain PspF 1−275 , or HrpRS, and in the presence (+) or absence (−) of HrpV (2 μM) and HrpG (2 μM). Gel images of transcripts for Figure 2a–e are shown in Supplementary Figure 4 . 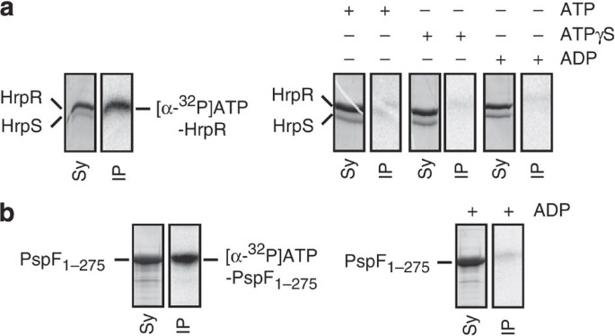Figure 4: ATP binding to HrpR and HrpS subunits. SDS–PAGE gel of ultraviolet radiated proteins. (a) Co-purified HrpRS in the presence of [α-32P]ATP and when supplemented with excess of non-labelled competitor nucleotides (as indicated). The relative concentrations of the Hrp proteins were visualized using SYPRO Ruby protein staining (Sy), and were compared with the relative intensities of the crosslinked radioactive species (determined by PhosphoImager analysis; IP). Full gel images are shown inSupplementary Figure 5. (b) As inausing PspF1−275as comparative control, for which specific ATP-binding methodology has been established39,45. ( f ) A bar graph showing electrophoretic mobility shifted hrpL DNA promoter probe comprising UAS sequences (in percentage of total hrpL DNA promoter signal) in the presence of HrpRS (2.5 μM) or HrpRS (2.5 μM and HrpV (4.2 μM). ( g ) A bar graph depicting the percentage of DNA bound in the closed promoter complex (CC) and transcriptionally proficient open promoter complex (OC; formed by PspF activation) in the presence of HrpRS–V or HrpV. ( h ) A bar graph depicting the relative amount of glutaraldehyde crosslinked HrpRS–HrpV species in either ATPase buffer (used to measure the ATPase activity of HrpRS+/−HrpV) or HGNED buffer. The relative amount of crosslinked HrpS–V complex was determined by fluorescence scanning. In f – h , estimated errors of measurements are shown as ±10%. Full size image Purified HrpV inhibited HrpRS-dependent activation of σ 54 -RNAP transcription ( Fig. 2d ) at a 1:1 ratio (HrpV:HrpRS), independent of the constant concentrations of DNA, σ 54 -RNAP and IHF. We infer that HrpV directly acts to diminish productive interactions HrpRS makes with the closed promoter complex. To establish that HrpV specifically inhibits the action of the HrpRS complex, we tested whether HrpV could inhibit transcription activation by an alternate EBP (the AAA+ domain of PspF), using the σ 54 -dependent Sinorhizobium meliloti nifH test promoter, which lacks the HrpRS UASs present in the hrpL promoter. As shown in Figure 2e , although PspF and HrpRS are both able to activate σ 54 -dependent transcription at the nifH promoter, only the activity of HrpRS is inhibited by HrpV. Clearly, the action of HrpV is specific in targeting HrpRS and does not require the UAS sequences (in line with the observation that HrpV does not reduce HrpRS UAS binding; ( Fig. 2f and see below). Moreover, the addition of HrpV or HrpRS–V did not destabilize preformed PspF-dependent σ 54 -RNAP OCs, suggesting HrpV acts before OC formation ( Fig. 2g ; compare OC to OC+HrpRS–V and OC+HrpV). HrpV did not inhibit the ATPase activity of HrpRS (where the ATPase turnover rate per min for 1 μM HrpRS was: 0.180±0.02 (minus HrpV), 0.192±0.02 (plus 1 μM HrpV) and 0.183±0.02 (plus 10 μM HrpV) and the ATPase buffer did not prevent HrpS from interacting with HrpV, Fig. 2h ). Overall, these data establish that HrpV acts via a mechanism specific to the HrpS subunit of the HrpRS complex, not previously described for other EBPs. Further, HrpG when added to the HrpRS–V regulatory complex ( Fig. 2e ), relieved some of the inhibitory action of HrpV (as observed in vivo ) but had no stimulatory effect on transcription activation by PspF. These results establish that HrpG functions as a specific suppressor for HrpV activity and that HrpG and HrpV can function independently of any Ps -specific factors. HrpRS co-dependency is hrpL promoter independent We established that the hrpL promoter (P hrpL ) contains a functional UAS between positions −147 to −36 relative to the transcription start-site ( Fig. 3a,b ), to which purified HrpR, HrpS and HrpRS bind in electrophoretic mobility shift assays ( Fig. 3c,d ). Consistent with the in vitro observations, in which addition of IHF greatly stimulated transcription ( Fig. 2a ), hrpL -dependent in vivo transcription in an IHF deletion strain was marginal ( Fig. 3b ). The specific IHF-binding site is present in the promoter probe ( Fig. 3e ), probably promoting productive interactions between HrpRS and σ 54 -RNAP, as evidenced by the increased transcription activity in vivo ( Fig. 3b ) and in vitro ( Fig. 2a ). Compared with either HrpR alone or HrpS alone or when HrpR and HrpS were mixed together (denoted as HrpR+HrpS, Fig. 3c ), co-purified HrpRS bound the UAS DNA with greater affinity ( Fig. 3d ), indicating co-operative binding to the P hrpL . Lack of increased UAS binding in the presence of pre-mixed, separately purified HrpR and HrpS, probably reflects incompetent subunit assembly (in line with the in vitro transcription assays; Fig. 2b ). 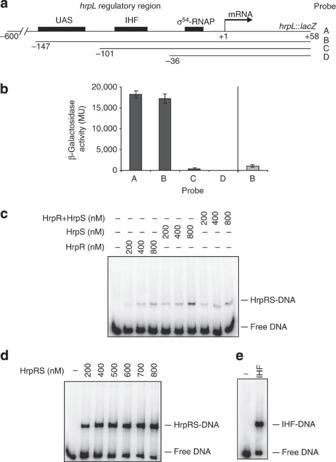These features of the hrpL promoter are in good agreement with other EBP interactions at σ 54 -dependent promoters in terms of co-operative binding to the UAS and exclude promoter architecture as the major basis of HrpRS co-dependency [43] . Figure 3:hrpLpromoter functional UAS site mapping and promoter binding. (a) Overview of upstream promoter truncation constructs of thehrpLpromoter DNA::lacZrepoter gene (A: −600 to +58; B: −147 to +58; C: −101 to +58 and D: −36 to +58; numbering with respect to the transcription start-site, +1) used to map functional UAS sequences and showing candidate UAS upstream activator sequences (black boxes), IHF (integration host factor) and σ54-RNAP-binding sites. (b)In vivotranscription from reporter constructs shown ina, in either wild-typeE.coli(MC4100, black bars) or an isogenic strain deleted for IHF coding sequence (grey bar). (c) Electrophoretic mobility shift assay using thehrpLpromoter probe with increasing HrpR, HrpS, pre-mixed HrpR and HrpS (HrpR+HrpS) concentrations (as indicated). (d) As incwith co-expressed, co-purified HrpRS (HrpRS). (e) Electrophoretic mobility shift assay of thehrpLpromoter probe with (10 nM) IHF. Inb, all assays were minimally performed in triplicate and standard errors of the mean are shown. Figure 3: hrpL promoter functional UAS site mapping and promoter binding. ( a ) Overview of upstream promoter truncation constructs of the hrpL promoter DNA:: lacZ repoter gene (A: −600 to +58; B: −147 to +58; C: −101 to +58 and D: −36 to +58; numbering with respect to the transcription start-site, +1) used to map functional UAS sequences and showing candidate UAS upstream activator sequences (black boxes), IHF (integration host factor) and σ 54 -RNAP-binding sites. ( b ) In vivo transcription from reporter constructs shown in a , in either wild-type E.coli (MC4100, black bars) or an isogenic strain deleted for IHF coding sequence (grey bar). ( c ) Electrophoretic mobility shift assay using the hrpL promoter probe with increasing HrpR, HrpS, pre-mixed HrpR and HrpS (HrpR+HrpS) concentrations (as indicated). ( d ) As in c with co-expressed, co-purified HrpRS (HrpRS). ( e ) Electrophoretic mobility shift assay of the hrpL promoter probe with (10 nM) IHF. In b , all assays were minimally performed in triplicate and standard errors of the mean are shown. Full size image HrpR and HrpS are not equivalent for nucleotide binding Identical subunits in EBPs and other AAA+ proteins make delineation of mechanistic roles of individual subunits experimentally challenging [44] . To directly probe any non-equivalence of HrpR and HrpS subunits (as suggested by the mutagenesis studies; Fig. 1c,d ), in the context of the purified functional HrpRS complex, we tested nucleotide binding with non-equilibrium covalent ultraviolet crosslinking [39] , [45] of [α- 32 P]ATP using PspF as a control. Recall that the highly conserved Walker A motif (GXXXXGK[T/S]), especially, the 'K' residue, is strictly required for nucleotide binding in AAA+ proteins [46] , including EBPs [39] , [47] . As shown in Figure 4 , HrpR and HrpS were separated by SDS–PAGE and the relative protein concentrations evaluated by SYPRO ruby protein stain fluorescence (Sy). The relative amount of [α- 32 P]ATP crosslinked protein species was determined by PhosphorImager analysis. Side-by-side comparison of the relative [α- 32 P]ATP/fluorescence intensities ( Fig. 4a ) of the HrpR and HrpS bands indicate that [α- 32 P]ATP preferentially crosslinks to HrpR and at a level comparable to that of the structurally and functionally characterized EBP PspF [39] ( Fig. 4b ). Specific binding of [α- 32 P]ATP to HrpR is further demonstrated by the competitive binding of non-radiolabelled ADP, ATP and ATPγS ( Fig. 4a ). Differential nucleotide binding to particular subunits of the strictly co-dependent HrpRS system provides direct evidence for non-equivalent nucleotide-dependent roles for individual subunits in a functional EBP complex. Figure 4: ATP binding to HrpR and HrpS subunits. SDS–PAGE gel of ultraviolet radiated proteins. ( a ) Co-purified HrpRS in the presence of [α- 32 P]ATP and when supplemented with excess of non-labelled competitor nucleotides (as indicated). The relative concentrations of the Hrp proteins were visualized using SYPRO Ruby protein staining (Sy), and were compared with the relative intensities of the crosslinked radioactive species (determined by PhosphoImager analysis; IP). 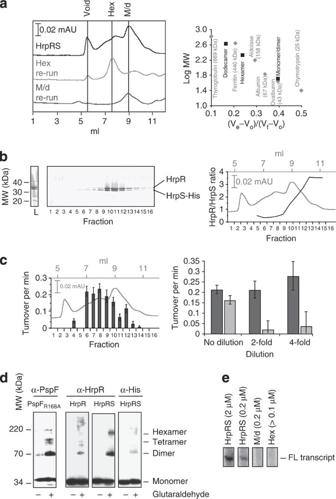Figure 5: A stable HrpRS hetero-hexameric species appears to be the active form. (a) Analytical HPLC gel-filtration vertically offset chromatograms of co-purified HrpRS (top); re-chromatographed fraction 7 (Hex re-run) and fraction 10 (monomer/dimer (M/d) re-run). The apparent monomer/dimer (m/d), hexamer (hex), void volume (void) retentions are indicated. Molecular mass standards (right) and their retention volumes used to calculate the apparent MW of the peaks. (b) SDS–PAGE of the SYPRO-stained fractions collected during gel-filtration ina. The relative fluorescence intensity ratios of HrpR/HrpS are plotted in the line graph (superimposed on the gel-filtration profile of HrpRS; grey). (c) Bar chart illustrating the ATPase turnover rates (min−1) of the fractions inb(superimposed on the gel-filtration profile of HrpRS; grey). Concentration-independent ATP turnover rates in a twofold dilution series of fraction 7 (hex) compared with dilutions of fraction 10 (m/d). (d) Glutaraldehyde crosslinked HrpR, HrpRS and PspFR168Acomplexes were separated by SDS–PAGE and analysed by western blotting using antibodies specific to HrpR (α-HrpR), HrpS (α-His) or PspF (α-PspF). Migration mobilities of several higher-order oligomeric species (labelled dimer, tetramer and hexamer) are indicated. (e)In vitrotranscription assay (as inFig. 2a, where FL represents the full-length transcript of∼470 nt) of the monomer/dimer fraction 10 froma(m/d) at 0.2 μM compared with an equimolar concentration of HrpRS (0.2 μM), before gel filtration. Inc, all assays were minimally performed in triplicates and standard errors of the mean are shown. Full gel images are shown in Supplementary Figure 5 . ( b ) As in a using PspF 1−275 as comparative control, for which specific ATP-binding methodology has been established [39] , [45] . Full size image The HrpRS hetero-hexamer is the most active assembly Gel-filtration of co-purified HrpRS ( Fig. 5a ) resolved at least two distinct species with molecular weights (MWs) corresponding to 212 kDa (apparent 6.1 mer) and 52 kDa (apparent 1.4 mer)—where the MW of HrpR is 34.9 kDa and HrpS His is 34.5 kDa. The lower MW peak does not permit assignment of subunit composition(s) and may comprise a mixture of monomers and dimers. SDS–PAGE analysis ( Fig. 5b ) of the fractions demonstrates that HrpR and HrpS are present in both peaks. Interestingly, we note that the relative intensities of HrpR and HrpS differ significantly between the hexameric (hex) species (where HrpS predominates over HrpR) and monomer/dimer species (where HrpR predominates over HrpS). The relative HrpR/HrpS fluorescence intensities are consistently scored as ∼ 0.5 in fractions 5–8; suggesting a fixed HrpR/HrpS stoichiometry in the hexameric fractions—although precise determination of the stoichiometry of this complex was not possible using this approach. Re-produced retention volumes ( Fig. 5a , hex re-run) and concentration-independent ATPase turnover rates of the re-chromatographed or diluted hexameric HrpRS fraction ( Fig. 5c ; fraction 7) indicate that the HrpRS hexamer is stable minimally over the purification and assay time course and at the concentrations used. Further evidence that HrpRS forms a mixed subunit hexameric assembly was obtained using glutaraldehyde protein–protein crosslinking ( Fig. 5d ); where a hexameric crosslinked species that reacted to HrpR- (α-HrpR) and His-tag-antibodies (to detect HrpS; α-His) was detected. Figure 5: A stable HrpRS hetero-hexameric species appears to be the active form. ( a ) Analytical HPLC gel-filtration vertically offset chromatograms of co-purified HrpRS (top); re-chromatographed fraction 7 (Hex re-run) and fraction 10 (monomer/dimer (M/d) re-run). The apparent monomer/dimer (m/d), hexamer (hex), void volume (void) retentions are indicated. Molecular mass standards (right) and their retention volumes used to calculate the apparent MW of the peaks. ( b ) SDS–PAGE of the SYPRO-stained fractions collected during gel-filtration in a . The relative fluorescence intensity ratios of HrpR/HrpS are plotted in the line graph (superimposed on the gel-filtration profile of HrpRS; grey). ( c ) Bar chart illustrating the ATPase turnover rates (min −1 ) of the fractions in b (superimposed on the gel-filtration profile of HrpRS; grey). Concentration-independent ATP turnover rates in a twofold dilution series of fraction 7 (hex) compared with dilutions of fraction 10 (m/d). ( d ) Glutaraldehyde crosslinked HrpR, HrpRS and PspF R168A complexes were separated by SDS–PAGE and analysed by western blotting using antibodies specific to HrpR (α-HrpR), HrpS (α-His) or PspF (α-PspF). Migration mobilities of several higher-order oligomeric species (labelled dimer, tetramer and hexamer) are indicated. ( e ) In vitro transcription assay (as in Fig. 2a , where FL represents the full-length transcript of ∼ 470 nt) of the monomer/dimer fraction 10 from a (m/d) at 0.2 μM compared with an equimolar concentration of HrpRS (0.2 μM), before gel filtration. In c , all assays were minimally performed in triplicates and standard errors of the mean are shown. Full size image Taking the relative total HrpRS protein concentrations of the individual gel filtered fractions into account, we determined the ATPase turnover rates of all fractions and found that the hexameric species was the most active ( Fig. 5c ). The HrpRS concentration in the hexameric fraction was too low to detect transcription in vitro ( Fig. 5e ). However, the gel-filtration purified HrpRS monomer/dimer fraction (fraction 10) was unable to detectibly activate σ 54 -RNAP, whereas the original loading sample (diluted to the same concentration as the gel-filtered HrpRS monomer/dimer fraction) supported transcription ( Fig. 5e ). We infer that the hexameric HrpRS assembly is the active form. These results suggest that a defined subunit composition of a HrpRS hexamer confers the highest transcription and ATPase activities. Gene duplication events followed by recombination and/or diversification are thought to be the major driving force for evolutionary innovation [48] , but knowledge of the molecular mechanisms that underpin selection of duplicated genes is fragmented [49] . Despite considerable hrp / hrc gene similarities, the evolution of hrpRS through duplication is the most distinguishing feature of Ps PAIs (pathovars include tomato, tagetis (marigold), phaseolicola (bean) and oryzae (rice)). We now provide insights into the mechanistic diversification of HrpR and HrpS and their regulation by HrpV and HrpG. Uncommon for gene duplication events, duplication of an EBP ancestor has not resulted in functional independence, but has locked the diverging HrpR and HrpS subunits into strict co-dependence, possibly explaining their high sequence conservation. HrpR appears to have become specialized in nucleotide-dependent functionalities, whereas HrpS retained a HrpV-dependent regulatory function. Our results suggest no obvious mechanistic advantage of the HrpRS system in activating σ 54 -dependent transcription when compared with singly acting EBPs, rather there may be regulatory advantages conferred by having only HrpS targeted by HrpV. In line with this, deletion of Lon protease correlates with HrpR (and not HrpS) accumulation in vivo —although it is unclear whether Lon degrades HrpR directly [16] , [17] , [19] . The divergent roles of HrpR and HrpS described here provide one example of regulatory specialization of one subunit of a strictly co-dependent system, thus illustrating how partial sub-functionalization (for example, reduced ATP binding by HrpS, inability of HrpR to interact with HrpV) could occur in combination with neo-functionalization (for example, acquisition of a novel interaction between HrpR and Lon) [19] . Purified HrpRS is competent to activate transcription, is negatively regulated in trans by HrpV and this repression is released by HrpG, establishing that the HrpRSVG system is sufficient for regulated expression at the hrpL promoter in vitro . Activity of HrpRS in E. coli , with K. pneumoniae σ 54 and S. meliloti promoter sequences indicated that the HrpRS system does not require Ps -specific factors to function. Amino-acid residues essential for nucleotide binding and hydrolysis are important for HrpRS activity in vivo , particularly in the case of HrpR. However, as the ATPase activity and oligomeric states have not been tested in vivo , we cannot exclude that assembly defects account for lack of activity. Significantly, mutations in catalytic residues in HrpS (D107, E108 and R226), thought essential for activity in EBPs, did not abolish transcription activity in HrpRS [39] , [50] . The requirement for both HrpR and HrpS σ 54 -binding motifs suggests an active, and not merely structural role, for each protein in the HrpRS complex. Binding of HrpV to HrpS and not HrpR implies a subunit-specific negative control mechanism not previously described for other EBPs. HrpV can completely repress HrpRS activity, but does not directly inhibit each subunit of the functional hexamer; potentially acting allosterically and/or sterically blocking access to the RNA polymerase closed complex. Allostery could be achieved through topological effects on the HrpRS hexameric ring in line with HrpV-mediated changes in the interactions between HrpR and HrpS (suggested in the BACTH assays; Fig. 1h ). The action of HrpV is distinct in that it does not alter the ATPase or DNA-binding activities of HrpRS. In contrast, NifL diminishes the ATPase and DNA-binding properties of the EBP NifA, and PspA inhibits the ATPase activity of PspF [11] , [51] . Heteromeric AAA+ proteins have been reported as stacked homo-hexameric rings (for example, the bacterial proteases ClpA/ClpX [52] and human ATPases Tip48/Tip49 (ref. 53 )), or as a single hetero-hexameric ring (in the case of eukaryotic MCM; Mcm2-7p), or as homo-multimers (as in prokaryotic and archeal MCM) [14] , [15] . Notably, the six distinct subunits of Mcm2-7p demonstrate clear mechanistic specialization in binding and hydrolyzing ATP [15] . We now show that HrpRS forms a hetero-hexameric structure. The distinct ATP-binding activities and functional roles of HrpR and HrpS provide direct evidence that individual subunits in EBPs may not be functionally equivalent, and that asymmetric functioning may underpin their action. Bacterial strains and plasmids FL hrpR , hrpS , hrpRS (as a single operon) , hrpV and hrpG genes were amplified by PCR from Ps DC3000 genomic DNA (see Supplementary Table S3 for all strains and plasmids used in this study). The bacterial two-hybrid (BACTH) fusion proteins were amplified with flanking 5′- XbaI and 3′- KpnI restriction sites and cloned into the corresponding pUT18C and pKT25 vectors. To construct the pUT18C- hrpS / hrpV plasmid (co-expressing T18-HrpS and WT HrpV) a DNA fragment encompassing the Shine–Dalgarno sequence and hrpV was PCR amplified to include flanking 5′- KpnI and 3′- E co RI restriction sites and cloned into pUT18C- hrpS (see Fig. 1g ). Mutations in hrpR or hrpS were introduced using the QuikChange method (Agilent technologies) as instructed. All recombinant plasmids were verified by sequencing. The P hrpL transcriptional lacZ -reporter fusion ( hrpL ∷ lacZ ) was constructed by amplifying 0.6 kbp of the hrpL promoter region as an EcoRI - BamHI fragment from Ps DC3000 genomic DNA and subcloning into pRS415 (ref. 54 )—creating pAVM415. The single-copy chromosomal fusion of hrpL ∷ lacZ was constructed as described [55] . Briefly, phage λBDC531 ( imm 21 ) was grown in a strain carrying pAVM415. The resulting λ phages were used to generate lysogens in SA1943 and screened for a Gal − phenotype on MacConkey galactose agar plates supplemented with ampicillin (100 μg ml −1 ). P1 phage was grown on the lysogens and the resultant lysates used to transduce the recipient strain DY226, which was screened for ampicillin resistant transductants at 42 °C. The constructed strain carrying the P hrpL ∷ lacZ fusion was then screened for the Bio + phenotype and the presence of prophage (sensitivity to λ phages). Finally, the P hrpL ∷ lacZ fusion was moved by P1 transduction (by selecting for ampicillin resistance) into strain MC4100, generating strain MJ2806. In vivo β-galactosidase assays β-Galactosidase assays [56] and BACTH assays were performed as described [32] . Briefly, proteins were fused to either the T18 or T25 fragments of adenylate cyclase (plasmids pT18C and pT25, respectively) and co-transformed into BTH101 cells. Interaction efficiencies were quantified by measuring the β-galactosidase activity of the cultures following induction (for 2 h at 25 °C) with 0.5 mM isopropyl-β- D -thiogalactoside at mid-log phase [56] . Protein purification Proteins used in this study, HrpR, HrpS, HrpRS, HrpV, HrpG, IHF, E. coli PspF, Kp σ 54 and Ps σ 54 , were over-expressed (using 0.5 mM isopropyl-β- D -thiogalactoside) in E. coli and purified essentially as described [25] . Briefly, cell pellets were re-suspended in buffer A NI (50 mM sodium phosphate buffer pH 7.0, 500 mM NaCl, 0.1 mM EDTA, 5% glycerol) supplemented with protease inhibitor cocktail (Roche), disrupted by sonication and the resultant soluble fraction purified by metal affinity chromatography using a linear gradient of 0–1 M imidazole (in buffer A NI ). The desired protein fractions were dialysed overnight against storage buffer (20 mM Tris pH 8.0, 50 mM NaCl, 0.1 mM EDTA and 5% glycerol). HrpG was purified from the insoluble cell fraction by urea-denaturation, which involved resuspending the cell pellet in buffer A NI containing 8 M urea. The rest of the Ni-affinity purification protocol remained the same. IHF was purified exactly as described [57] . FL transcription assays FL transcription assays were performed in either TTH (10 mM Tris-HCl, pH 7.5, 70 mM KCl, 5 mM MgCl 2 , 1 mM dithiothreitol, 1 mM EDTA, 12.5% glycerol and 0.1% w/v Triton X-100) or STA (25 mM Tris-acetate, pH 8.0, 8 mM Mg-acetate, 10 mM KCl and 3.5% w/v PEG 6000) buffer (for the hrpL or nifH promoters respectively) in a 10 μl volume containing 100 nM σ 54 -RNAP (reconstituted at a 1:5 ratio RNAP:σ 54 ), 20 nM supercoiled promoter DNA and where stated 4 mM dATP, 20 nM IHF and equimolar (to [HrpRS]) concentrations of HrpV and/or HrpG (unless stated). OC formation was initiated by addition of 0.8 μM HrpR, HrpS or HrpRS (for the hrpL promoter, unless otherwise stated) or 2 μM HrpRS or PspF (for the nifH promoter, unless otherwise stated) and incubated at room temperature (RT) for 1 h. Concentration stated refers to the monomer concentration for HrpR, HrpS or PspF and the dimer concentration for HrpRS. Transcription was initiated with a mix containing 100 μg ml −1 heparin, 0.1 mM ATP, CTP, GTP, 0.05 mM UTP and 3 μCi of [α- 32 P]UTP and incubated for 10–20 min at RT ( hrpL ) or 37 °C ( nifH ). Reactions were quenched with loading dye and analysed on 6% denaturing gels. Gels were dried and transcripts visualized and quantified using a Fuji FLA-5000 PhosphorImager. In vitro glutaraldehyde crosslinking Assays were conducted in a total reaction volume of 10 μl, in HGNED buffer (25 mM HEPES, pH 8.0, 1 mM dithiothreitol, 100 mM NaCl, 0.2 mM EDTA, 0.05% (v/v) NP-40 and 10% (v/v) glycerol) containing 2.5 μM of the specified proteins. Samples were treated with glutaraldehyde (at a final concentration 0.1%) and incubated at RT for 10 min. Reactions were stopped by addition of 2 μl stop solution (200 mM Tris-HCl pH 7.5, 200 mM glycine). Crosslinked protein complexes were separated by 10% SDS–PAGE and analysed by western blotting (see below). Western blotting Crosslinked complexes were separated by SDS–PAGE and transferred onto polyvinylidene difluoride membrane using a semidry transblot system (Bio-Rad). Western blotting was performed as described [11] using antibodies specific to either Ps HrpR (α-HrpR; 1:10,000), Ps HrpS (α-HrpS; 1:10,000), Ps HrpV (α-HrpV; 1:5,000), E. coli PspF (α-PspF; 1:4,000), His-tag (to detect HrpS; α-His; 1:1,000; Promega) or the BACTH fusion construct pKT25 (α-pKT25; 1:500). Proteins were detected using the ECL plus Western Blotting Detection Kit (GE Healthcare) as instructed. In vitro native gel mobility shift assays Assays were performed in TTH (see above) buffer in a 20 μl total reaction volume at RT. Briefly, 10 nM of a 32 P-end labelled DNA fragment (comprising the −147 to +58 region of the hrpL promoter: relative to the transcription start-site, +1) was incubated with 0.8 μM of either HrpR, HrpS or co-expressed HrpRS and, where indicated, HrpV and/or IHF at the specified concentrations (see figure legends). All reactions were incubated at RT for 15 min and protein–DNA complexes resolved by 4.5% native-PAGE. The gels were dried and complexes visualized and quantified using a Fuji FLA-5000 PhosphorImager (Fuji). ATP binding and hydrolysis assays ATP binding was carried out in 20 μl total reaction volume containing 10 μM of purified protein in reaction buffer (20 mM Tris pH 8.0, 50 mM NaCl, 0.1 mM EDTA and 5% glycerol)) supplemented with 40 μCi [α- 32 P] ATP (3,000 Ci mmol −1 ). Sample drops were spotted onto a 4 °C cooled glass plate and exposed to ultraviolet light, illuminating (254 nm, UVG-54, UVP) for 15 min on ice. Reactions were stopped by adding 10 μl formic acid and proteins resolved by 12% SDS–PAGE analysis. Gels were stained by Sypro-ruby fluorescent protein stain (Invitrogen) and protein band intensities visualized and quantified on Fuji FLA-5000 as instructed by the supplier (Bio-Rad). Then gels were dried and radioactivity visualised and quantified by phospho-imaging (Fuji FLA-5000 with Tina 2.10g software). ATPase assays were conducted in ATPase reaction buffer (20 mM Tris pH 8.0, 50 mM NaCl, 0.1 mM EDTA and 5% glycerol), incubated for 1 h at 22 °C with 100 μM ATP containing 0.06 μCi μl −1 [α- 32 P] ATP. Proteins were at a final concentration of 10 μM. Reactions were stopped by adding 5 volumes of 2 M formic acid. Released [α- 32 P] ADP was separated from ATP by thin layer chromatography and radiolabelled [α- 32 P]-ADP and [α- 32 P]-ATP quantified by phospho-imaging (Fuji FLA-5000). ATPase assays were also performed in the nifH buffer system (which permits HrpV-dependent inhibition of HrpRS transcription activation activity), omitting the dATP and substituting this for 100 μM ATP—illustrating that the inability of HrpV to repress HrpRS ATPase activity is not simply due to unfavourable buffer conditions [39] . Gel-filtration assays Gel-filtration chromatography was carried out at RT in running buffer (20 mM Tris pH 8.0, 50 mM NaCl, 15 mM MgCl2, 0.02% (w/v) azide) at a 0.7 ml min −1 flow rate using a BioCad Sprint HPLC system and a Bio-Sep-S 3000 column (Phenomenex), as described previously [58] . The column was calibrated using MW standards (Sigma): Blue Dextran (200 kDa), Thyroglobulin (669 kDa), Ferritin (440 kDa), Catalase (232 kDa), Aldolase (158 kDa), Albumin (67 kDa), Ovalbumin (43 kDa), Chymotrypsin (25 kDa) and Ribonuclease (13.5 kDa). Fractions were analysed by SDS–PAGE using SYPRO ruby stain (Invitrogen) and quantified using a Fuji FLA-5000 fluorescence reader. M.J. prepared most constructs, designed, carried out and analysed all in vivo work (transcription, BACTH, UAS mapping, IHF); performed to in vitro transcription with hrpL, EMSA, including IHF purification and contributed to writing of Materials and Methods. E.H.J. worked on the evolution, purification of HrpRS, HrpV and HrpG; HrpG work and analysis; contributed to editing manuscript and contributed to writing of Materials and Methods. P.C.B. designed and established the heterologous in vitro transcription assay, including abortive conditions and linear DNA probes, collated and prepared figures for publication and contributed significantly to editing manuscript. F.G.M.R. purified HrpRS and carried out DNA binding and gluaraldehyde crosslinking experiments and also purified Ps σ 54 for in vitro transcription experiments and contributed to writing of Materials and Methods. M.B. conceived the project design and experimental approaches, oversaw the study, interpretations of data and writing of the manuscript. J.S. designed, carried out and analysed in vitro work (ATPase, gel filtration, ultraviolet crosslinking), conceived the evolution work, contributed to the project design, oversaw the study, interpreted data and wrote the manuscript. How to cite this article: Jovanovic, M. et al . Regulation of the co-evolved HrpR and HrpS AAA+ proteins required for Pseudomonas syringae pathogenicity. Nat. Commun. 2:177 doi: 10.1038/ncomms1177 (2011).